Identification of a potent palladium-aryldiphosphine catalytic system for high-performance carbonylation of alkenes The development of stable and efficient ligands is of vital significance to enhance the catalytic performance of carbonylation reactions of alkenes. Herein, an aryldiphosphine ligand ( L11 ) bearing the [Ph 2 P(ortho-C 6 H 4 )] 2 CH 2 skeleton is reported for palladium-catalyzed regioselective carbonylation of alkenes. Compared with the industrially successful Pd/1,2-bis(di-tert-butylphosphinomethyl)benzene catalyst, catalytic efficiency catalyzed by Pd/ L11 on methoxycarbonylation of ethylene is obtained, exhibiting better catalytic performance (TON: >2,390,000; TOF: 100,000 h −1 ; selectivity: >99%) and stronger oxygen-resistance stability. Moreover, a substrate compatibility (122 examples) including chiral and bioactive alkenes or alcohols is achieved with up to 99% yield and 99% regioselectivity. Experimental and computational investigations show that the appropriate bite angle of aryldiphosphine ligand and the favorable interaction of 1,4-dioxane with Pd/ L11 synergistically contribute to high activity and selectivity while the electron deficient phosphines originated from electron delocalization endow L11 with excellent oxygen-resistance stability. Carbonylation of alkenes via transition metal catalysis provides a straightforward and atom-efficient approach to synthesis carboxylate and its derivatives [1] , [2] , [3] , [4] , [5] , which represent important structural scaffolds in the pharmaceutical, polymer, cosmetics, food industries [6] , [7] , [8] , [9] . Various catalytic systems based on palladium, rhodium, nickel, copper and cobalt have been developed, and Pd/phosphine complexes exhibit outstanding catalytic performance under more mild reaction conditions [5] , [10] , [11] , [12] , [13] , [14] . Due to the critical role of phosphine ligands for controlling catalytic activity and selectivity on alkoxycarbonylation of alkenes, it is highly significant to design efficient phosphine ligands and elucidate how they can modulate the catalytic performance. In the past decades, several phosphine ligands have been developed, exhibiting good catalytic activity and selectivity on alkoxycarbonylation of alkenes. In the 1990s, 1,2-bis(di-tert-butylphosphinomethyl)benzene (DTBPMB) was developed for palladium-catalyzed methoxycarbonylation of ethylene, producing methyl propionate (MP) with 100,000 of TON and 12,000 h −1 of TOF, which provides the basis to synthesize the fundamental methyl methacrylate via the Lucite’s Alpha process (Fig. 1 ) [15] , [16] , [17] . This versatile DTBPMB ligand was also applied to alkoxycarbonylation of aliphatic alkenes with high selectivity for linear esters and acids [18] , [19] . Moreover, great efforts on designing alkyl phosphines with bulky steric substituents have been devoted for controlling the activity and selectivity of alkoxycarbonylation of alkenes, such as, bis(di-tert-butylphosphanyl)benzene [20] , [21] and bis(diphosphaadmantyl)alkanes [22] . Nevertheless, these catalytic systems are still limited with the unsatisfactory reaction performance and inferior ligand stability. Recently, Beller’s group designed two ligands containing both tertiary butyl and pyridyl groups on the P-atom, 1,2-bis((tert-butyl(pyridin-2-yl)phosphanyl)methyl)benzene (py t bpx) and 1,1’-bis(tert-butyl(pyridin-2-yl)phosphanyl)ferrocene (py t bpf), achieving better catalytic efficiency with 1,425,000 of TON and 44,000 h −1 of TOF on methoxycarbonylation of ethylene (Fig. 1 ) [23] , [24] , [25] . Despite these state-of-the-art systems, the above-mentioned alkyl phosphines still suffer from drawbacks such as expensive cost and easy oxidation. From the point of view of both academia and industry, it is highly desirable to develop a stable and potent phosphine ligand that is efficient, inexpensive, practically operated, and resistant to air. Fig. 1: Ligand advances in palladium-catalyzed carbonylation of alkenes. TON turnover number, TOF turnover frequency, DTBPMB 1,2-bis(di-tert-butylphosphinomethyl)benzene, py t bpx 1,2-bis((tert-butyl(pyridin-2-yl)phosphanyl)methyl)benzene, py t bpf 1,1’-bis(tert-butyl(pyridin-2-yl)phosphanyl)ferrocene. Full size image As known, aryl phosphines are more stable toward oxidation due to better electron delocalization compared to the aliphatic counterparts. However, aryl phosphines normally afford lower activity than alkyl ones in alkoxycarbonylation of alkenes [17] , [23] , [26] , [27] , [28] . On the other hand, the bite angle (P-M-P) of diphosphine ligands coordinated with metal centers has been elucidated to be vital for the modulation of activity and selectivity because the energy barriers of key transition state and intermediates during the catalytic cycle can be regulated by changing the electronic structure and steric hindrance [29] , [30] . In alkoxycarbonylation, the electron density of metal center decreases with the bite angle of P-M-P increasing, thus facilitating nucleophilic attack of the alcohols and methanolysis of acyl palladium species [19] , [31] . However, the chelation ability is weakened with excessive large bite angle, leading to low catalytic performance [26] , [29] . Therefore, the appropriate P-Pd-P bite angle is beneficial for acquiring high reactivity on alkoxycarbonylation of alkenes. [Ph 2 P(ortho-C 6 H 4 )] 2 CH 2 has been developed as one of the most attractive skeletons of aryldiphosphine ligands where the aryl phosphine can rotate within limits owing to the presence of [CH 2 ], leading to inherent but limited flexibility and optimal coordination mode with the metal center [32] , [33] . It can be speculated that the [Ph 2 P(ortho-C 6 H 4 )] 2 CH 2 skeleton incorporating appropriate substituents might provide the sweet P-Pd-P bite angle for alkoxycarbonylation of alkenes with high catalytic performance. As such, it has resulted in a call for developing [Ph 2 P(ortho-C 6 H 4 )] 2 CH 2 based aryldiphosphine ligands with appropriate bite angle and electron delocalization enabling high catalytic performance. However, no efficient aryl phosphine ligand has ever been reported up to now. Herein, we demonstrate an example of highly stable and efficient aryldiphosphine ligand based on [Ph 2 P(ortho-C 6 H 4 )] 2 CH 2 skeleton for palladium-catalyzed carbonylation of alkenes. Compared with the reported py t bpx and industrially applied DTBPMB ligand, our aryldiphosphine ligand not only exhibits better catalytic performance (TON: >2,390,000; TOF: 100,000 h −1 ; selectivity: >99%), but also presents stronger oxygen-resistance stability (over 100 days of exposure under air), thus providing a potential application (1000 ppm of oxygen tolerance) for industrial production (Fig. 1 ). Catalytic performance study Initially, a variety of representative diphosphine ligands were screened when using methoxycarbonylation of 1-octene and methanol as the benchmark reaction (Fig. 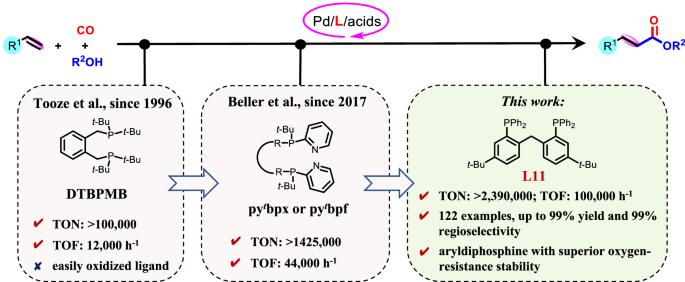Fig. 1: Ligand advances in palladium-catalyzed carbonylation of alkenes. TON turnover number, TOF turnover frequency, DTBPMB 1,2-bis(di-tert-butylphosphinomethyl)benzene, pytbpx 1,2-bis((tert-butyl(pyridin-2-yl)phosphanyl)methyl)benzene, pytbpf 1,1’-bis(tert-butyl(pyridin-2-yl)phosphanyl)ferrocene. 2a and Supplementary Table 1 ). In the presence of state-of-the-art industrial ligand DTBPMB ( L1 ), 83% yield and 92% regioselectivity were obtained under methanol as previous literature reported [18] , [19] , but difficult to actuate the transformation at all when using 1,4-dioxane. This peculiar phenomenon demonstrated that 1,4-dioxane inhibited the Pd/ L1 -catalyzed methoxycarbonylation. Other DTBPMB-type ligands ( L2 and L3 ) replacing the alkyl tert-butyl groups by aryl rings exhibited low yields and regioselectivities. Besides, aryldiphosphine ligands DPPB ( L4 ) and DPPN ( L5 ) with rigid skeletons showed no activity at all. However, Xantphos ( L6 ) showed 6% yield and 82% regioselectivity. Interestingly, a semi-rigid aryldiphosphine ligand ( L7 ) with inherent but limited flexibility promoted methoxycarbonylation of 1-octene with 41% yield and 86% regioselectivity. The conversion and selectivity were further improved by replacing the [O] linkage with [CH 2 ] group ( L8 ) with 44% yield and 91% regioselectivity, thus inspiring us to modify this [Ph 2 P(ortho-C 6 H 4 )] 2 CH 2 scaffold. Ligands bearing various aryl substitutes ( L9 - L11, L13 and L14 ) were tested and tertiary butyl group modified aryldiphosphine ligand L11 offered the optimal activity (66%) and regioselectivity (91%). However, with more flexible aryldiphosphine ligand L12 , no activity was observed on the methoxycarbonylation of 1-octene. With the optimal aryldiphosphine ligand L11 , influences of the solvents and other reaction parameters were investigated (Supplementary Tables 2 – 6 , Supplementary Fig. 12 , and Fig. 2a ). Finally, the yield and regioselectivity were further improved up to 95% and 91%, respectively, under the optimal reaction condition: 0.2 mol% Pd(acac) 2 , 0.8 mol% L11 , 2 mol% TsOH·H 2 O, in 4 ml 1,4-dioxane, 2 MPa CO, 100 °C for 20 h. Fig. 2: Ligand optimization and its application in methoxycarbonylation. a Ligand optimization for methoxycarbonylation of 1-octene; Reaction condtions: 1-octene (2 mmol), methanol (8 mmol), Pd(acac) 2 (0.2 mol%), L (0.8 mol%), TsOH·H 2 O (2 mol%), CO (2 MPa), 1,4-dioxane (4 ml), 100 °C, 3 h, GC yields of the mixture of linear and branched esters are based on 1-octene using n-decane as the internal standard, the ratio of linear and branched esters is determined by GC analysis and is shown in parentheses; a Methanol (4 ml) instead of 1,4-dioxane as the solvent; b 1-octene (8 mmol), methanol (2 mmol), 20 h. b Methoxycarbonylation of ethylene at mole-scale; Reaction conditions: ethylene (2.0 mol), methanol (1200 ml), Pd(acac) 2 (0.00069 mmol), L11 (0.5 mmol), TsOH·H 2 O (4.0 mmol), CO (8.0 MPa), 100 °C, 48 h for TON, or 18 h for TOF. TON, turnover number. TOF, turnover frequency. py t bpx, 1,2-bis((tert-butyl(pyridin-2-yl)phosphanyl)methyl)benzene. Full size image Methyl propionate commercially produced by Pd 2 (dba) 3 / L1 -catalyzed methoxycarbonylation of ethylene is the starting material to synthesize methyl methacrylate (MMA), which is the important unit of polymethylmethacrylate (PMMA) generally applied in biomedicine, sensors, battery electrolytes, molecular separations, polymer conductivity, and ect [34] , [35] . Herein, the methoxycarbonylation of ethylene at mole-scale was successfully performed in presence of L11 even when the Pd dosage decreased to 0.33 ppm (Fig. 2b , Supplementary Figs. 13 and 14 ), affording prominent activity (TON: >2,390,000; TOF: 100,000 h −1 ) and selectivity (>99%). Remarkably, this Pd(acac) 2 / L11 catalytic system demonstrated higher catalytic efficiency than the optimal Pd(acac) 2 /py t bpx (TON: >1,425,000; TOF: 44,000 h −1 ; selectivity: >99%) and Pd 2 (dba) 3 / L1 (TON: >100,000; TOF: 12,000 h −1 ; selectivity: >99%) catalytic systems reported so far [17] , [24] , thus providing more promising industrial application of this catalytic system. Investigation of the oxygen-resistance stability The oxygen-resistance stability comparison between L11 and L1 was examined (Fig. 3 ). After being exposed under air at room temperature, the phosphine atom on L1 was quickly oxidized after several days, whereas the pristine phosphine valence state of L11 was still unchanged even after 100 days of exposure (Fig. 3 a, b, and Supplementary Figs. 15 and 16 ). Afterwards, the methoxycarbonylation of 1-octene was conducted under different oxygen contents in presence of Pd/ L11 and Pd/ L1 , respectively. Notably, the activities were increased gradually as the oxygen content decreased from 10000 to 1 ppm when using Pd/ L11 system in dioxane, and 25% yield was achieved even at 1000 ppm of oxygen content while no yield was observed for Pd/ L1 system even at 1 ppm (Fig. 3c , and Supplementary Fig. 17 ). Because methanol was a common-used solvent in the state-of-the-art Pd/ L1 system, thus the oxygen-resistance stability was also tested in methanol. 48% yield was observed using Pd/ L11 in presence of 1000 ppm of oxygen content whereas only trace amount of the desired product was obtained using Pd/ L1 (Fig. 3d and Supplementary Fig. 18 ). Importantly, the reaction solution displayed transparent yellow after methoxycarbonylation catalyzed by Pd/ L11 in the case of 1,4-dioxane or methanol as a solvent, whereas palladium black particles were observed obviously using Pd/ L1 under identical reaction conditions (Supplementary Figs. 19 and 20 ). Fig. 3: Comparison tests of oxygen-resistance stability between L1 and L11. a , b Stability tests of L1 and L11 under air conditions at room temperature, respectively. c , d Stability tests of L1 and L11 during the reaction process in 1,4-dioxane or methanol, respectively. e Change in Gibbs’ free energy (∆G r ) for L1 and L11 oxidation, computed at DFT level. f HOMO orbitals of L1 and L11 . Full size image Density functional theory (DFT) calculations revealed that the Gibbs’ free energy (∆G r ) upon oxidation for L11 was less negative than that for L1 (−203.3 vs −222.3 kJ/mol, Fig. 3e ), and the energy difference between HOMO orbital of L11 and LUMO orbital of triplet oxygen was larger than that of L1 (235.85 kJ/mol vs 222.48 kJ/mol), indicating L11 was more resistant to oxidation than L1 . Furthermore, the electron orbital in L11 spanned larger range than that in L1 , showing that the stronger electron delocalization of L11 was the intrinsic factor resistant to the oxidation (Fig. 3f ). These comparison results demonstrated that aryldiphosphine ligand L11 possessed stronger oxygen-resistance stability for both storage and reaction, which was crucial for its practicability due to the possible reduction of industrial operating costs. Mechanism study The relationship between the bite angle of P-Pd-P and the catalytic activity was investigated (Fig. 4b ). The yield of methoxycarbonylation of 1-octene improved rapidly as increasing the bite angle of P-Pd-P from 87.62° ( L4 ) to 99.68° ( L11 ), and then declined sharply with the ligand bite angle further increased from 99.68° ( L11 ) to 113.90° ( L12 ). The highest activity was obtained in presence of L11 , indicating that appropriate bite angle of P-Pd-P around 100° was benificial for achieving the highest catalytic activity. Owing to the rate-limitation role of methanolysis of acyl palladium species (min3 to product) (Fig. 4a ), the correlation between the activation energy of this elementary step and activity was examined (Fig. 4c ) [25] . The yield of methoxycarbonylation of 1-octene slipped from 66% to 0% as the values of ∆G(min3 to product) increased from −4.1 to 4 kJ/mol. Subsequently, the dependence between bite angle of P-Pd-P and ∆G was explored where the minimal value of ∆G (−4.1 kJ/mol) was obtained in presence of L11 (Fig. 4d ). So, it could be concluded that aryldiphosphine ligand L11 with appropriate bite angle of P-Pd-P was responsible for the optimal catalytic activity because of the lowest energy barrier of min3 to product. Fig. 4: Investigation of the ligand bite angel and solvent effect. a Computed structure of R, TS, min, and P, and plausible mechanism. b Dependence between bite angles of P-Pd-P and yield of methoxycarbonylation of 1-octene. c Dependence between △ G(min3 to product) and yield of methoxycarbonylation of 1-octene via various aryldiphosphine ligands. d Dependence between bite angles of P-Pd-P and △ G(min3 to product). e Experimental tests and Boltzmann populations of the selected solvents on solvent effect. f Free energy profiles for the formation of linear (L; blue) and branched esters (B; red); See Fig. 4a for the computed structure of R, TS, min, and P. g DFT optimized structures of the initial complex with 1,4-dioxane (highlighted in yellow), [PdH( L11 )(dioxane)] + , and upon hydride insertion to 1-butene (highlighted in pink), [PdH( L11 )(dioxane)(butene)] + -L, [PdH( L11 )(dioxane)(butene)] + -B; Legend of colors: White (H), Gray (C), Red (O), Orange (P), and Petrol Green (Pd). Full size image When using 1,4-dioxane, methanol, and anisole in methoxycarbonylation of 1-octene, 91%, 74%, and 86% regioselectivities were obtained, respectively, while no activity was observed at all when reacting in acetonitrile and 1,2-dimethoxyethane (Fig. 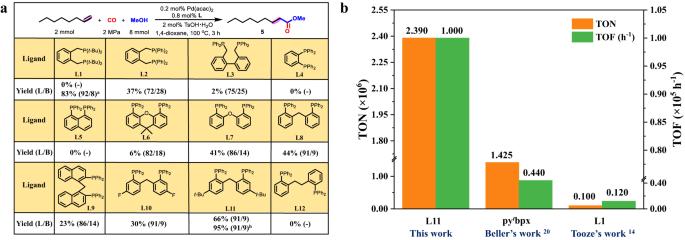Fig. 2: Ligand optimization and its application in methoxycarbonylation. aLigand optimization for methoxycarbonylation of 1-octene; Reaction condtions: 1-octene (2 mmol), methanol (8 mmol), Pd(acac)2(0.2 mol%), L (0.8 mol%), TsOH·H2O (2 mol%), CO (2 MPa), 1,4-dioxane (4 ml), 100 °C, 3 h, GC yields of the mixture of linear and branched esters are based on 1-octene using n-decane as the internal standard, the ratio of linear and branched esters is determined by GC analysis and is shown in parentheses;aMethanol (4 ml) instead of 1,4-dioxane as the solvent;b1-octene (8 mmol), methanol (2 mmol), 20 h.bMethoxycarbonylation of ethylene at mole-scale; Reaction conditions: ethylene (2.0 mol), methanol (1200 ml), Pd(acac)2(0.00069 mmol),L11(0.5 mmol), TsOH·H2O (4.0 mmol), CO (8.0 MPa), 100 °C, 48 h for TON, or 18 h for TOF. TON, turnover number. TOF, turnover frequency. pytbpx, 1,2-bis((tert-butyl(pyridin-2-yl)phosphanyl)methyl)benzene. 4e and Supplementary Table 2 ). Then, DFT calculations were conducted to reveal the origin of regioselectivity. The overall pathway of alkoxycarbonylation of alkenes can be formally divided into three consecutive steps: (1) hydride insertion to alkene (R → TS1 → min1), (2) coordination and insertion of CO (min1 → min2 → TS2 → min3), and (3) methanolysis (min3 → TS3 → P) (Fig. 4a ), where the hydride insertion to alkene was the key step in determining the regioselectivity [1] , [36] . The energy files for the reaction pathways of linear and branched products in different solvents were illustrated (Fig. 4f and Supplementary Fig. 21 ). Clearly, the differences of ∆G a between TS1(B) and TS1(L) during the hydride insertion to alkene in 1,4-dioxane was 1.2 kJ/mol, higher than that in MeOH (0.8 kJ/mol) and anisole (0.7 kJ/mol), confirming that the linear reaction pathway in 1,4-dioxane was more kinetically favored. The relative ratios for the L/B in 1,4-dioxane methanol, and anisole were also calculated by Boltzmann population to be 89%, 80% and 84%, respectively, which matched well with the experimental data, further proving the hydride insertion to alkene determined the regioselectivity (Fig. 4e ). Under the optimal catalytic system, the coordination chemistry of 1,4-dioxane with Pd/ L11 was crucial for determining the regioselectivity. Compared with other solvents, a specific interaction between the oxygen lone-pair electrons of 1,4-dioxane and a hydrogen atom of the phenyl rings of L11 was verified with a distance of 2.393 Å, leading to an in situ formed configuration of [PdH( L11 )(1,4-dioxane)] + (R) (Fig. 4g ). This interaction was the reason leading to the highest ∆G a difference (1.2 kJ/mol) between TS1(B) and TS1(L) during the hydride insertion to 1-butene, indicating the preferable formation of the TS1(L). The highest ∆G a difference probably arisen from the steric hindrance of TS1(B) configuration, leading to the high regioselectivity towards linear product. However, ∆G a of the hydride insertion to alkene for acetonitrile or 1,2-dimethoxyethane was too high to initiate the catalytic cycle (Supplementary Fig. 21 ), suggesting their reaction paths were kinetically hindered. Consequently, the specific 1,4-dioxane effect benefited the linear reaction pathway, thus enhancing the selectivity towards the linear esters [37] , [38] , [39] . Subsequently, various control experiments were conducted to gain mechanistic insight into the reaction. The crude solution after 0.5 h of methoxycarbonylation of 1-octene was investigated and subjected to run the high-resolution mass spectrometry analysis. An assignable peak located at m/z = 853.2495 was observed, which was attributed to Intermediate A (Supplementary Fig. 22 ; chemical formula: C 50 H 53 O 2 P 2 Pd + , exact mass: 853.2550). This result indicated that the formed Intermediate A might be involved in the proposed catalytic cycle. Furthermore, in situ generated Pd-P intermediates were also detected in methoxycarbonylation of 1-octene by [31] P NMR measurements (Supplementary Figs. 23 and 24 ). Remarkably, chemical shifts of the Pd-P intermediates before and after reaction changed from 24.05 to 20.90 ppm, attributing to in situ generated [PdH( L11 )(1,4-dioxane)] + (R) [40] . In situ high-pressure FTIR analysis was conducted to monitor the dynamic catalytic behavior of the Pd/ L11 and other intermediates during the reaction process (Supplementary Fig. 25 ). 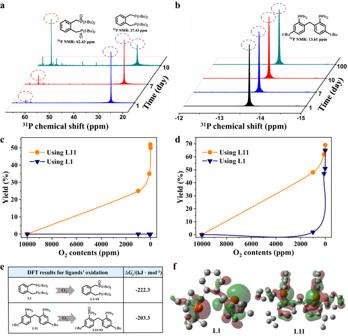Fig. 3: Comparison tests of oxygen-resistance stability between L1 and L11. a,bStability tests ofL1andL11under air conditions at room temperature, respectively.c,dStability tests ofL1andL11during the reaction process in 1,4-dioxane or methanol, respectively.eChange in Gibbs’ free energy (∆Gr) forL1andL11oxidation, computed at DFT level.fHOMO orbitals ofL1andL11. With the reaction temperature increasing from 30 to 100 °C, characteristic peaks of the Pd-H (palladium–hydride) and Pd-P (palladium–phosphine) species, both of which were identified as the key active intermediates that made the catalytic reaction proceeding smoothly, appeared immediately at 1929 and 970 cm −1 , respectively, and then reached its maximum intensities at about 100 °C (Supplementary Fig. 25b, c ) [41] . The peaks at 2017, 1988, and 1971 cm −1 were assigned to vibrations of Pd-CO that were the complexation results of various Pd/ L11 intermediates with CO (Supplementary Fig. 25b ) [42] , [43] . Furthermore, two peaks at 3078 and 1640 cm −1 were ascribed to the stretching vibration of =C-H and -C=C- on 1-octene, and these signal intensities became weaken with the reaction temperature rising (Supplementary Fig. 25a, b ); meanwhile, the signal intensity of stretching vibration of -C=O- of the target ester located at 1739 cm −1 was intensified, which demonstrated the consumption of 1-octene and the generation of methyl nonanoate as the reaction process goes on. These mechanism studies confirmed that the Pd-P and Pd-H intermediates were active species during the catalytic process and formation of which were facilitated in the presence of L11 . Scope of the methodology Substrate compatibility of common alkenes and alcohols for alkoxycarbonylation or hydroxycarbonylation was tested (Fig. 5 ). Both short- ( 1 – 3 ) and long-chain ( 4 – 6 ) aliphatic alkenes were converted to the desired linear esters smoothly, affording excellent yields (84–97%) and regioselectivities (74–91%). Aliphatic alkenes with bulky steric hindrance groups ( 7 and 8 ) were well tolerated with excellent regioselectivities (92-99%) because the large steric hindrance groups inhibited the branched step of hydride insertion to alkene. Notably, alkene ( 9 ) bearing both internal and terminal C=C bonds reacted selectively at the position of terminal C=C bond, obtaining 89% yield and 97% regioselectivity. Moreover, aliphatic alkenes with chlorine ( 10 ), ketone ( 11 ), and ester ( 12 and 13 ), and chiral aliphatic alkene ( 14 ) were equally applicable. Importantly, diesters 15 to 19 , which has potential applications in polymer chemistry, were also directly synthesized with up to 80% yield and 85% regioselectivity through methoxycarbonylation of terminal dienes. Furthermore, various aryl alkenes ( 20 – 26 ), allylbenzenes ( 27 – 28 ), and allyl phenyl sulfone ( 29 ) were also employed and afforded the desired esters in good to excellent yields (51–96%) and regioselectivities (83-96%). Fig. 5: Substrate scope of common alkenes and alcohols. Detailed experimental procedures and reaction parameters for the various substrates were included in Supplementary Information. Full size image Primary ( 30, 31, 33 , and 37 ) and secondary ( 32, 34, 36, 38 and 39 ) aliphatic alcohols were converted to the corresponding esters in nearly quantitative yields and excellent regioselectivities. Comparatively, tertiary aliphatic alcohol afforded the target ester ( 35 ) with lower yield (41%) and regioselectivity (85%) because the hydroxycarbonylation of 1-octene was occurred due to the formation of H 2 O caused by the dehydration of tertiary amyl alcohol. Besides, aliphatic alcohols ( 40 – 42 ) bearing terminal alkene, ether, or ester group were converted smoothly to give linear esters with up to 97% yield and 92% regioselectivity. Gratifyingly, this catalytic system also allowed efficient multi-alkoxycarbonylations of polyhydric alcohols for direct synthesis of plasticizers and polyol ester base oil [44] , [45] , [46] , producing the corresponding polyesters ( 43 – 45 ) with excellent yields (86–99%) and regioselectivities (75–86%). Thiocarbonylations of thiols were also realized to yield the corresponding thioesters ( 46 – 48 ) with up to 84% yield and 93% regioselectivity. Subsequently, versatile benzyl alcohol derivatives ( 49 – 63 ) were investigated to the afford desired esters with up to 99% yield and 92% regioselectivity. Other aryl-substituted and heteroaromatic alcohols were also well tolerated, affording up to 99% yield and 91% regioselectivity ( 64 – 69 ). 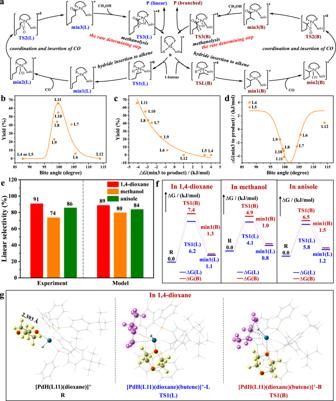Fig. 4: Investigation of the ligand bite angel and solvent effect. aComputed structure of R, TS, min, and P, and plausible mechanism.bDependence between bite angles of P-Pd-P and yield of methoxycarbonylation of 1-octene.cDependence between△G(min3 to product) and yield of methoxycarbonylation of 1-octene via various aryldiphosphine ligands.dDependence between bite angles of P-Pd-P and△G(min3 to product).eExperimental tests and Boltzmann populations of the selected solvents on solvent effect.fFree energy profiles for the formation of linear (L; blue) and branched esters (B; red); See Fig.4afor the computed structure of R, TS, min, and P.gDFT optimized structures of the initial complex with 1,4-dioxane (highlighted in yellow), [PdH(L11)(dioxane)]+, and upon hydride insertion to 1-butene (highlighted in pink), [PdH(L11)(dioxane)(butene)]+-L, [PdH(L11)(dioxane)(butene)]+-B; Legend of colors: White (H), Gray (C), Red (O), Orange (P), and Petrol Green (Pd). Carboxylic acids which are widely applied in the synthesis of polymers, cosmetics, pharmaceuticals [47] , [48] , [49] , [50] , [51] , were also produced by hydroxycarbonylation of alkenes. Both aliphatic ( 70 to 78 ) and aromatic ( 79 to 82 ) carboxylic acids were generated with up to 99% yield and 99% linear regioselectivity. Notably, linear dicarboxylic acids ( 73 to 77 ), as desirable synthon in the manufacture of polymers (such as Nylon PACM-12), fragrances, lubricants [52] , [53] , were directly synthesized with good yields (68–80%) and regioselectivities (75–88%) via hydroxycarbonylation of terminal dienes, thus proving the wide practicality of this catalytic system. Next, methoxycarbonylation of internal alkenes were also conducted catalyzed by the presented Pd/ L11 catalytic system (Fig. 6 ). For aliphatic internal alkenes ( 83 – 85 ), remarkable activity (86–98%) and moderate linear regioselectivity (57-64%) of the desired products were achieved. Meanwhile, cyclic internal alkenes, such as cyclohexene ( 86 ), cycloctene ( 87 ), and norbornene ( 88 ), reacted smoothly to yield the corresponding esters with up to 97% yield and 100% selectivity. Aromatic internal alkene of β-methylstyrene ( 89 ) could also afford the target ester with 90% yield and 75% linear regioselectivity. Furthermore, aliphatic and aromatic branched alkenes ( 90 – 94 ) were also employed and afforded the corresponding linear esters in good to excellent yields (68–98%) and outstanding regioselectivities (>99%). Notably, methoxycarbonylation of industrially important 1,3-butadiene ( 95 ) could also proceed well, giving moderate reactivity and regioselecyivity toward the dimethyl adipate. Fig. 6: Substrate scope of internal and branched alkenes, as well as 1, 3-butadiene. Detailed experimental procedures and reaction parameters for the various substrates were included in Supplementary Information. Full size image The late-stage modification of lead compounds or even actual drugs is of current interest for the discovery of new bioactive agents [54] , [55] . To validate the practicality of this methodology, the late-stage functionalized bioactive or chiral alkenes and alcohols for alkoxycarbonylation or hydroxycarbonylation were investigated (Fig. 7 ). Alkenes derived from drugs or natural products, including formononetin ( 96 ), sesamol ( 97 ), coumarin ( 98 ), hymecromone ( 99 ) and estrone ( 100 ) functionalities were successfully converted to the corresponding esters in high efficiency (82–95% yields and 81–91% regioselectivities). The biomass-based alkenes, eugenol ( 101 ), and methyl 5-allyl-3-methoxysalicylate ( 102 ) were also eligible candidates as well. Moreover, bioactive alcohols, including (-)-menthol ( 103 ), L(-)-borneol ( 104 ), citronellol ( 105 ), piperonyl alcohol ( 106 ), (±)-methylmandelate ( 107 ), tryptophol ( 108 ), estradiol benzoate ( 109 ), dehydroepiandrosterone ( 110 ), diosgenin ( 111 ), and mesterolone ( 112 ), were employed to furnish the desired esters with 75–99% yields and 85–91% regioselectivities. Notably, hydroxycarbonylation of these alkenes from bioactive or chiral derivatives ( 113 – 119 ) generated the desire acids with up to 90% yield and 97% regioselectivity, further highlighting the potential synthetic utility of this protocol [56] . Fig. 7: Late-stage functionalization of bioactive alkenes and alcohols. Detailed experimental procedures and reaction parameters for the various substrates were included in Supplementary Information. Full size image Nandrolone phenylpropionate ( 120 ), trenbolone enanthate ( 121 ), and testosterone enanthate ( 122 ) were a class of anabolic hormone approved by FDA (Food and Drug Administration), which were commonly-used in drug therapy for the palliative treatment of women with advanced breast cancer, the ideal contraceptive of male, and the increase of muscle strength and circumference, respectively. Gratifyingly, gram-scale synthesis of these clinically important pharmaceutical molecules were realized directly by the alkoxycarbonylation of the corresponding alkenes and alcohols under this potent Pd/ L11 catalytic system, exhibiting excellent reaction performance ( 120 : 1.53 g, 94% yield, 87% linear selectivity; 121 : 1.39 g, 87% yield, 83% linear selectivity; 122 : 0.553 g, 72% yield, 92% linear selectivity) (Fig. 8 ). This application further validated the potential practicability of this protocol for the synthesis of pharmaceutical molecules. Fig. 8: Gram-scale synthesis of clinically important pharmaceutical molecules. Detailed experimental procedures and reaction parameters for the various substrates were included in Supplementary Information. Full size image In summary, a stable and efficient aryldiphosphine ligand with [Ph 2 P(ortho-C 6 H 4 )] 2 CH 2 skeleton for palladium-catalyzed regioselective carbonylation of alkenes was developed. With the optimal ligand L11 , higher catalytic efficiency was obtained on methoxycarbonylation of ethylene (TON: >2,390,000; TOF: 100,000 h −1 ; selectivity: >99%), which represented excellent catalytic performance so far and possessed stronger oxygen-resistance stability compared with the industrially successful Pd/DTBPMB catalyst. Various alkenes and alcohols were well tolerated and selectively transformed to the desired linear esters or acids with up to 99% yield and 99% regioselectivity. Importantly, the late-stage carbonylation of bioactive and chiral alkenes or alcohols were successfully achieved with high activity and regioselectivity; gram-scale synthesis of clinically important pharmaceutical molecules, nandrolone phenylpropionate, trenbolone enanthate, and testosterone enanthate were also realized via this protocol. Experimental and computational investigations indicated that the appropriate P-Pd-P bite angle of the Pd/ L11 and the favorable 1,4-dioxane effect with the Pd/ L11 synergistically improved the catalytic activity and regioselectivity. Moreover, electron deficient phosphines on aryldiphosphine ligand caused by the electron delocalization were responsible for better oxygen-resistance stability. General information All reactions involving air and water-sensitive materials were performed under argon atmosphere. All chemicals were purchased from Innochem, Energy Chemical, J&K Scientific, Sigma-Aldrich, Acros Organics and used without further purification unless otherwise noted. Analytical thin layer chromatography (TLC) was performed using pre-coated Jiangyou silica gel HSGF254 (0.2 mm ± 0.03 mm). Visualization of the developed chromatogram was performed by UV absorbance (254 nm) or TLC stains (KMnO 4 solution). Flash chromatography was performed using silica gel 60, 0.063–0.2 mm, 200–300 mesh (Jiangyou, Yantai) with the indicated solvent system. GC-MS analyses were performed with on an Agilent 5977 A MSD GC-MS. Gas chromatography analyses were performed on an Agilent 7890 A GC equipped with a HP-5 capillary column and FID detector. Nuclear magnetic resonance spectra were recorded on a Bruker AvanceTM III 400 MHz in deuterated chloroform unless otherwise noted. Data are reported in parts per million (ppm) as follows: chemical shift, multiplicity (s = singlet, d = doublet, t = triplet, q = quartet, quint = quintet, m = multiplet, dd = doublet of doublet and br = broad signal), coupling constant in Hz and integration. The high-resolution mass spectrometry was recorded on a Bruker Q-TOF II MSD. X-ray crystallographic analyses were performed on a Bruker Smart APEX II, all the crystal structure diagrams were drawn by the Ortep-3 program [57] . HPLC analysis for measuring values of linear/branched products was performed on a Waters-Breeze system (2487 Dual λ Absorbance Detector and 1525 Binary HPLC Pump). Chiralpak AD-H columns were purchased from Daicel Chemical Industries, LTD. All measurements were carried out at room temperature unless otherwise stated. In situ high-pressure FT-IR spectra were obtained using a Nicolet NEXUS 670 spectrometer, the spectral resolution was about 4 cm −1 . General procedure for alkoxycarbonylation or hydroxycarbonylation An 80 ml steel autoclave was charged with Pd(acac) 2 (1.2 mg, 3.94 μmol, 0.2 mol%), L11 (10.4 mg, 16.05 μmol, 0.8 mol%), TsOH·H 2 O (7.6 mg, 40.00 μmol, 2 mol%), and 1,4-dioxane (4 ml). Then alkenes (8 mmol) and alcohols or H 2 O (36 mg, 2 mmol) were introduced into the autoclave. After the autoclave was purged with CO (1 MPa) for four times at room temperature and then pressurized with CO to 2 MPa, the autoclave was sealed and put into a preheated reactor, stirring at 100 °C for 20 h. Afterwards, the autoclave was cooled to room temperature and depressurized slowly. 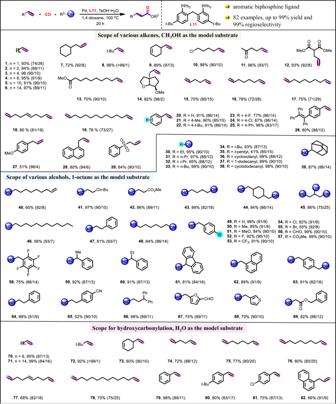Fig. 5: Substrate scope of common alkenes and alcohols. Detailed experimental procedures and reaction parameters for the various substrates were included in Supplementary Information. Subsequently, the reaction mixture was diluted with EtOAc (6.0 ml). Finally, the total yields of linear and branched esters or acids were obtained by gas chromatography analysis, flash column chromatography on silica gel, or acid-base extraction, and the regioselectivities of linear and branched esters or acids were obtained by gas chromatography analysis, liquid chromatography analysis, or 1 H NMR analysis. Detailed experimental procedures and reaction parameters for the various substrates were included in Supplementary Information. 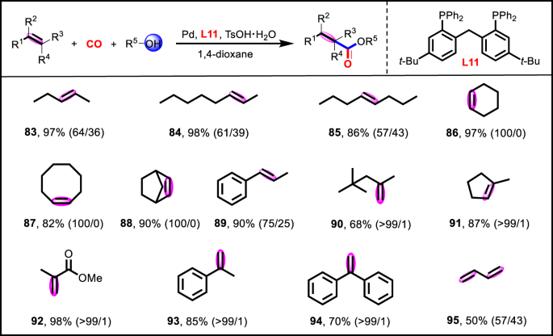Fig. 6: Substrate scope of internal and branched alkenes, as well as 1, 3-butadiene. Detailed experimental procedures and reaction parameters for the various substrates were included in Supplementary Information. Synthetic procedure of L11 A solution of n -butyllithium in hexane (2.5 M, 8.8 ml, 22 mmol) was added dropwise over a period of 10 min to a solution of bis(2-bromo-4-(tert-butyl)phenyl)methane (4.38 g, 10 mmol) in anhydrous tetrahydrofuran (60 ml) at −78 °C under argon atmosphere. 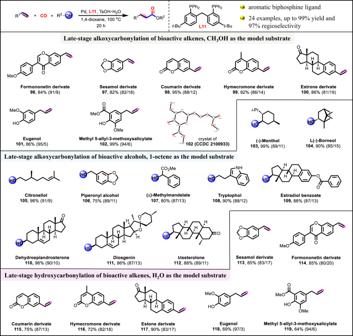Fig. 7: Late-stage functionalization of bioactive alkenes and alcohols. Detailed experimental procedures and reaction parameters for the various substrates were included in Supplementary Information. 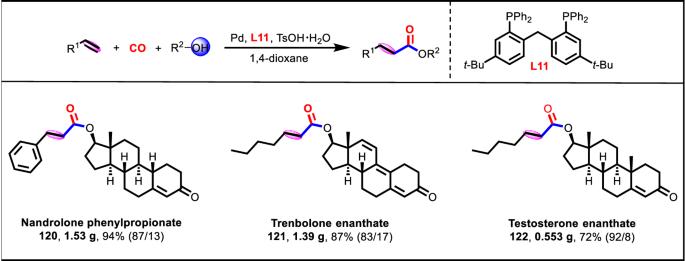Fig. 8: Gram-scale synthesis of clinically important pharmaceutical molecules. Detailed experimental procedures and reaction parameters for the various substrates were included in Supplementary Information. The solution was stirred for 1 h and then chlorodiphenylphosphine (4.84 g, 22 mmol) dissolved in anhydrous tetrahydrofuran (5 ml) was added dropwise. The mixture was continued to stir at −78 °C for 1 h and the system was heated to room temperature, and allowed to react overnight. The reaction was quenched with 2 N HCl solution. The mixture was extracted with ethyl acetate and water for 3 times, the combined organic phases were dried over anhydrous Na 2 SO 4 , and concentrated under reduced pressure. The residue was purified by flash column chromatography on silica gel using EtOAc–petroleum ether mixture (1:50) as an eluent to afford the desired compound L11 as a white solid (4.2 g, 65% yield). Caution: The usage of n -butyllithium in hexane should be careful and protected by inert atmosphere owing to its easy flammability under air or moisture condition. Detailed synthetic procedures and reaction parameters for the other ligands were included in Supplementary Information.